Increases in terrestrially derived carbon stimulate organic carbon processing and CO2emissions in boreal aquatic ecosystems The concentrations of terrestrially derived dissolved organic carbon have been increasing throughout northern aquatic ecosystems in recent decades, but whether these shifts have an impact on aquatic carbon emissions at the continental scale depends on the potential for this terrestrial carbon to be converted into carbon dioxide. Here, via the analysis of hundreds of boreal lakes, rivers and wetlands in Canada, we show that, contrary to conventional assumptions, the proportion of biologically degradable dissolved organic carbon remains constant and the photochemical degradability increases with terrestrial influence. Thus, degradation potential increases with increasing amounts of terrestrial carbon. Our results provide empirical evidence of a strong causal link between dissolved organic carbon concentrations and aquatic fluxes of carbon dioxide, mediated by the degradation of land-derived organic carbon in aquatic ecosystems. Future shifts in the patterns of terrestrial dissolved organic carbon in inland waters thus have the potential to significantly increase aquatic carbon emissions across northern landscapes. Emissions of carbon dioxide (CO 2 ) from inland waters to the atmosphere are now recognized as significant relative to other components of the Earth carbon system [1] , [2] , [3] , [4] . These emissions are fuelled by land-derived carbon [1] , [5] , [6] , and one of the pathways leading to widespread aquatic CO 2 supersaturation involves the transport of dissolved organic carbon (DOC) from land to continental waters and its subsequent degradation within the aquatic network. There is now mounting evidence that shifts in climate and other environmental factors are driving increasing aquatic concentrations of terrestrially derived DOC in many landscapes of the world [7] , [8] , [9] , in what has been termed the ‘browning’ [10] of inland waters. Whereas the magnitude and regulation of the browning phenomenon are the focus of intense research and debate [7] , [11] , [12] , [13] , [14] , [15] , [16] , [17] , the potential implications of such a shift in terrestrial carbon (C) concentrations for the functioning of the receiving aquatic systems have been less explored, particularly in terms of the impacts on aquatic CO 2 emissions. In this context, understanding the mechanistic underpinnings of the links between terrestrial DOC and aquatic CO 2 becomes critical to our ability to predict the potential impact of current and projected shifts in the delivery of this terrestrial carbon on global aquatic CO 2 emissions [18] . DOC and CO 2 concentrations are indeed positively related across temperate and boreal lakes [19] , [20] , [21] , [22] but the mechanisms underlying this relationship are still debated [19] . Should the positive relationship between CO 2 and DOC be mostly driven by the covariation between the loading of terrestrial DOC and that of soil-derived CO 2 , then the use of this relationship to understand and predict the effects of increasing DOC on surface water CO 2 dynamics is questionable. If, in contrast, the relationship between DOC and CO 2 is to a large extent driven by the actual degradation of terrestrially derived DOC into CO 2 within aquatic systems, then this relationship has a causal underpinning and can be used to predict future scenarios involving changes in the concentrations of terrestrial DOC in continental waters. Understanding the potential for the degradation of terrestrially derived DOC is therefore essential to establish the link between DOC and CO 2 dynamics. It has long been recognized that terrestrial DOC is susceptible to photochemical degradation in the water [23] , but it has traditionally been assumed that this DOC is generally recalcitrant to biological degradation [24] , [25] , [26] , and therefore that the contribution of this latter pathway to aquatic CO 2 production is modest. This view is rapidly changing [24] , [25] , and a growing volume of evidence indicates that terrestrial DOC may be readily degraded by biological processes in aquatic environments, such as the Amazon basin [27] and the Arctic [8] , [28] , temperate [29] , [30] and boreal [31] , [32] biomes. Boreal biomes contain the highest density of freshwater on Earth, yet this evidence for biologically degradable DOC is scattered and based on isolated components of the continental aquatic network. As a result, the overall susceptibility of DOC to photochemical and biological degradation, and how this susceptibility varies over gradients of increasing terrestrial influence and at scales relevant for continental C budgets, has not been well established [19] , [33] , [34] , [35] , [36] . Here we explicitly address the mechanistic underpinnings of the relationship between aquatic CO 2 and DOC and, in particular, we explore the concentrations of photochemically degradable DOC and Bd-DOC, and surface water CO 2 dynamics in boreal aquatic networks. We base this work on simultaneous measurements of Biologically degradable DOC and photochemically degradable DOC, as well as ambient CO 2 concentrations and fluxes, in hundreds of lakes, wetlands and rivers across the northern boreal landscapes of Québec (Canada), spanning a very large gradient of both DOC and terrestrial influence. We first assess how these two facets of DOC degradability vary along a gradient of increasing terrestrial influence (using chromophoric dissolved organic matter (CDOM) as a proxy (see Supplementary Note 1 ) and then explore to what extent DOC degradability mediates the relationship between terrestrial DOC and aquatic CO 2 concentrations and fluxes. Environmental gradients covered The conditions covered in this study encompass much of the range in environmental conditions reported in the literature for northern freshwaters ( Supplementary Table S1 ). In particular, surface water concentrations of DOC ranged from 2.1 to 123.9 mg l −1 (median=9.4 mg l −1 ) across all sites, and CDOM ranged from 0.13 to 30 m −1 (median=4.4 m −1 , absorption coefficient measured at 440 nm in Naperian units); both were strongly, positively correlated ( r 2 =0.60, Supplementary Fig. S1 ), suggesting that much of the variability in ambient DOC concentrations is driven by differences in the loading of terrestrial DOC. The vast majority of ecosystems was supersaturated in CO 2 (average partial pressure of CO 2 ( p CO 2 ) was 754, 3,396 and 5,896 μatm for lakes, rivers and wetlands, respectively), and thus emitted CO 2 to the atmosphere (average CO 2 flux was 450, 1,459 and 960 mg C m −2 d −1 for lakes, rivers and wetlands, respectively). DOC degradability patterns To reconstruct the links between terrestrial DOC and aquatic CO 2 fluxes, we first assessed the patterns in DOC degradability based on measurements of the amount of DOC lost to biological and photochemical processes under standardized conditions (see Methods). There were positive relationships between the amounts of both Biologically degradable DOC (Bd-DOC) and photochemically degradable DOC (Pd-DOC) and CDOM concentrations across lakes, wetlands and rivers ( Fig. 1 ). Although it could be a priori expected that higher amounts of degradable DOC would result from increasing overall amounts of DOC, it is the nature of the relationships reported here that is of particular interest. The slope of the type II regression (see Methods) between Bd-DOC and CDOM ( Fig. 1a ; log-slope=1.15, 95% confidence interval=0.97–1.35, P <0.001) indicates that across the whole gradient of systems studied, the DOC pool in the brownest systems with the highest terrestrial influence was as biologically degradable (in terms of the proportion that can be removed) as the DOC pool in clearer waters. In systems with higher terrestrial influence, DOC was in fact proportionately more photochemically degradable ( Fig. 1b ; log-slope=1.54, 95% CI=1.40–1.68, P <0.001). As a result, the percentage of Bd-DOC shows no significant relationship with CDOM ( P =0.82) but the percentage of Pd-DOC increases significantly with CDOM ( r 2 =0.30, P <0.0001, Supplementary Fig. S2 ). 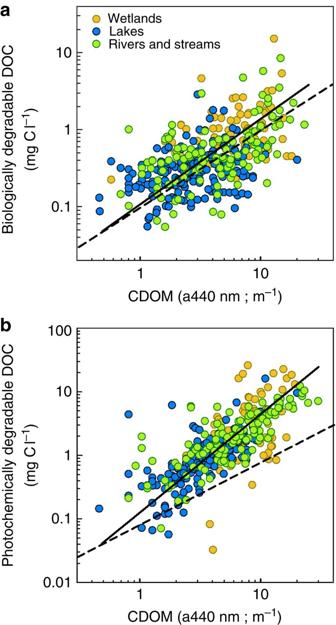Figure 1: Concentrations of degradable DOC across gradients of terrestrial influence. Concentrations of Bd-DOC and Pd-DOC increase as a function of ambient CDOM for natural water samples from a wide range of aquatic systems in the boreal and temperate landscapes of Québec, Canada. (a) Log(Bd-DOC)=1.15 Log(CDOM) (95% confidence interval (CI)=0.97–1.35); 1.00,P<0.0001,n=345,r2=0.30. (b) Log(Pd-DOC)=1.54 Log(CDOM)(95% CI=1.40–1.68); 0.90,P<0.0001,n=359,r2=0.59. The dashed lines represent a slope of 1, that is, a proportional increase in degradable DOC as CDOM increases. Figure 1: Concentrations of degradable DOC across gradients of terrestrial influence. Concentrations of Bd-DOC and Pd-DOC increase as a function of ambient CDOM for natural water samples from a wide range of aquatic systems in the boreal and temperate landscapes of Québec, Canada. ( a ) Log(Bd-DOC)=1.15 Log(CDOM) (95% confidence interval (CI)=0.97–1.35); 1.00, P <0.0001, n =345, r 2 =0.30. ( b ) Log(Pd-DOC)=1.54 Log(CDOM)(95% CI=1.40–1.68); 0.90, P <0.0001, n =359, r 2 =0.59. The dashed lines represent a slope of 1, that is, a proportional increase in degradable DOC as CDOM increases. Full size image Linking DOC processing to CO 2 dynamics Stable or increasing DOC degradability over gradients of terrestrial influence suggest that increasing CDOM should lead to enhanced conversion of DOC to CO 2 in aquatic ecosystems, and thus to higher concentrations and fluxes of CO 2 . There was indeed a positive relationship between ambient p CO 2 and CDOM across all our systems ( Supplementary Fig. S3 ), but whether or not this pattern may be directly attributed to the conversion of DOC to CO 2 within those systems cannot be determined by this simple relationship. Alternative mechanisms unrelated to direct DOC degradation, including the covariation in the loading of soil-derived DOC and CO 2 to aquatic systems, could also explain this relationship. To explicitly address these different scenarios, we further explored the causal links that may exist between terrestrially derived DOC, DOC degradability, and excess aquatic CO 2 concentrations and flux ( f CO 2 , in mg C m −2 d −1 ) using structural equation modelling (SEM) [37] . In addition to empirically determining the existence of a link between CDOM and f CO 2 , this approach allows to determine the pathways by which CDOM is most probably influencing CO 2 . We tested several alternative structures linking CDOM to CO 2 for all the sampled sites (see Supplementary Fig. S4 for key examples), and the only statistically significant structure is one where CDOM-related increases in both Bd-DOC and Pd-DOC positively influence aquatic p CO 2 , and subsequently aquatic f CO 2 ( Fig. 2a ). The two paths leading from CDOM to f CO 2 were highly significant, suggesting that both biological and photochemical processing of DOC contribute significantly to the observed CO 2 dynamics. Note that this structure did not contain a significant direct link between CDOM and p CO 2 , the latter reflecting variables that influence p CO 2 and that may co-vary with CDOM, such as soil-derived CO 2 . Interestingly, although there was a significant positive relationship between p CO 2 and DOC across all systems ( r 2 =0.28, P <0.001), there were no significant structures linking DOC, DOC degradability and CO 2 ( Supplementary Fig. S4 ), thus suggesting that it is the degradation of the terrestrial component of DOC (CDOM) that is more directly influencing aquatic CO 2 dynamics. 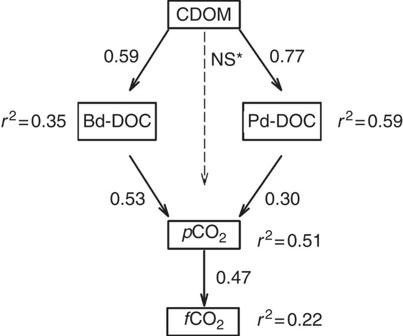Figure 2: Linking terrestrially derived DOC to aquatic fluxes of CO2. Structural equation model linking changes in aquatic CDOM to changes in CO2fluxes to the atmosphere. Arrows denote directional links between two variables, and the coefficients represent the rate at which a response variable varies as a function of a given change in its predictor, based on centered and standardized data (see Methods). All paths are significant atP<0.001. The dashed arrow denotes a non-significant (NS*) path that was not included in the final model presented here; it is included only for presentation purposes to emphasize the absence of a significant direct link between CDOM andpCO2or CO2flux.pCO2represents excesspCO2. Degradation-mediated CDOM indirect effect coefficient onfCO2is 0.25.n=216.χ2=5.20,P=0.39, df=5. Figure 2: Linking terrestrially derived DOC to aquatic fluxes of CO 2 . Structural equation model linking changes in aquatic CDOM to changes in CO 2 fluxes to the atmosphere. Arrows denote directional links between two variables, and the coefficients represent the rate at which a response variable varies as a function of a given change in its predictor, based on centered and standardized data (see Methods). All paths are significant at P <0.001. The dashed arrow denotes a non-significant (NS*) path that was not included in the final model presented here; it is included only for presentation purposes to emphasize the absence of a significant direct link between CDOM and p CO 2 or CO 2 flux. p CO 2 represents excess p CO 2 . Degradation-mediated CDOM indirect effect coefficient on f CO 2 is 0.25. n =216. χ 2 =5.20, P =0.39, df=5. Full size image The effect of physical forcing While Fig. 2 suggests an important role of DOC processing for aquatic CO 2 dynamics, it also shows that at this scale, the regulation of CO 2 dynamics is not homogenous across all systems. Roughly half of the variation in p CO 2 was explained by factors other than DOC degradation, and, considering that fluxes are a direct function of concentration, the relationship between excess p CO 2 and f CO 2 was unexpectedly weak ( r 2 =0.22). Physical forcing, however, strongly mediates the p CO 2 versus f CO 2 relationship, with low-turbulence (expressed by the gas exchange coefficient, k CO2 in m d −1 ) sites sustaining higher average CO 2 concentrations for a given CO 2 production or input rate than systems that typically have higher turbulence [38] . In this regard, there was a clear bimodal distribution of the empirically determined k CO2 around a median of 1 m d −1 across all sampled sites ( Fig. 3a ), and the regression of f CO 2 against p CO 2 drastically improved when sites with k CO2 over and below 1 m d −1 were considered separately ( Fig. 3b ). This suggests that, at the expense of the generality of the relationship presented in Fig. 2 , separating sites into more homogenous groups with regard to physical structure provides a more robust quantification of the impact of changing terrestrial DOC concentrations on aquatic CO 2 fluxes. 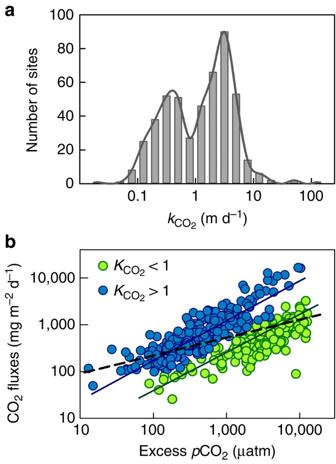Figure 3: Relationship between concentrations and fluxes of CO2. (a) Frequency distribution of the measured diffusivekCO2across the sampled sites. Note the bimodal distribution aroundkCO2=1 m d−1. (b) Regression of CO2fluxes to the atmosphere as a function of surface water CO2excess partial pressure for systems withkCO2over and below 1. Analysis of covariance reveals different intercepts (P<0.001) but similar slopes (P=0.08) for both groups.kCO2>1: Log(fCO2)=0.73 (±0.03) Log(excess CO2)−0.77 (±0.08),n=247,P<0.0001,r2=0.74.kCO2<1: Log(fCO2)=0.73 (±0.03)Log(excess CO2)−0.26 (±0.13),n=172,P<0.0001,r2=0.68. Dashed line illustrates the inadequacy of an overall fit in the absence of grouping: Log(fCO2)=0.36 (±0.03)Log(excess CO2)+1.67 (±0.09),n=419,P<0.001,r2=0.27. Note that sample size differs here compared withFigs 2and4, hence the different coefficients of determination betweenpCO2andfCO2. Figure 3: Relationship between concentrations and fluxes of CO 2 . ( a ) Frequency distribution of the measured diffusive k CO2 across the sampled sites. Note the bimodal distribution around k CO2 =1 m d −1 . ( b ) Regression of CO 2 fluxes to the atmosphere as a function of surface water CO 2 excess partial pressure for systems with k CO2 over and below 1. Analysis of covariance reveals different intercepts ( P <0.001) but similar slopes ( P =0.08) for both groups. k CO2 >1: Log( f CO 2 )=0.73 (±0.03) Log(excess CO 2 )−0.77 (±0.08), n =247, P <0.0001, r 2 =0.74. k CO2 <1: Log( f CO 2 )=0.73 (±0.03)Log(excess CO 2 )−0.26 (±0.13), n =172, P <0.0001, r 2 =0.68. Dashed line illustrates the inadequacy of an overall fit in the absence of grouping: Log( f CO 2 )=0.36 (±0.03)Log(excess CO 2 )+1.67 (±0.09), n =419, P <0.001, r 2 =0.27. Note that sample size differs here compared with Figs 2 and 4 , hence the different coefficients of determination between p CO 2 and f CO 2 . Full size image Quantifying the effect of CDOM on CO 2 fluxes On the basis of above results, we repeated the SEM analysis separately for these two subgroups of sites that were split based on their k CO2 (sites below and above 1 m d −1 , Fig. 4 ). The structures that emerged as significant for each separate group generally resembled that obtained for the ensemble of data shown in Fig. 2 , but there were some differences in the resulting links and parameters with implications for the prediction of aquatic CO 2 emissions. As mentioned above, there was no significant direct link between CDOM and p CO 2 when all the systems are considered ( Fig. 2 ), suggesting that the effect of CDOM on p CO 2 at the whole-network scale is predominantly degradation mediated. This direct link became significant, however, when high and low k CO2 systems were analysed separately, implying that a fraction of the CDOM effect was not due to DOC degradation when more homogenous groups of sites were considered. Moreover, the path connecting Pd-DOC and p CO 2 was non-significant in low-turbulence systems ( Fig. 4a ). As a result, most of the overall CDOM effect on f CO 2 (0.39, Fig. 4b ) was mediated by Bd-DOC and Pd-DOC (combined coefficient=0.30, Fig. 4b ) for high k CO2 systems (mostly lakes and fast-flowing rivers), while roughly half (coefficient=0.20, Fig. 4a ) of the overall CDOM effect on f CO 2 (coefficient=0.37) was not mediated by either Bd-DOC or Pd-DOC for low k CO2 systems (mostly wetlands and slow-flowing rivers). These coefficients can then be used to estimate how CO 2 fluxes respond to increases in CDOM and, together, the different SEM analyses thus provide insights on the links that exist between terrestrial influence and CO 2 emissions in aquatic ecosystems, in particular, on the role that DOC processing plays in that framework. 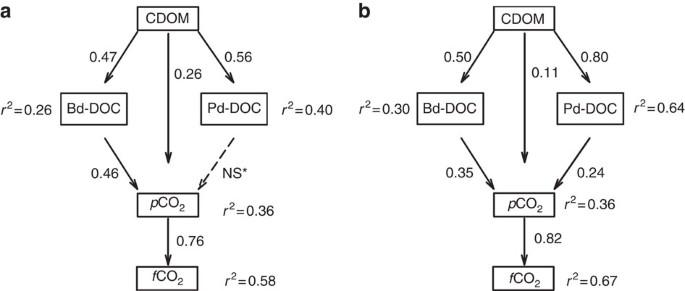Figure 4: The pathways linking CDOM to CO2fluxes in high- and low-turbulence systems. Structural equation models linking changes in aquatic CDOM to changes in CO2fluxes to the atmosphere for the two subsets of sites separated on the basis ofkCO2and therefore of average turbulence. Arrows denote directional links between two variables, and the coefficients represent the rate at which a response variable varies as a function of a given change in its predictor, based on centered and standardized data (see Methods). All paths are significant atP<0.001. The dashed arrow denotes a non-significant (NS*) path that was not included in the final model presented here; it is included only for presentation purposes to emphasize the absence of a significant direct link between Pd-DOC andpCO2in low-turbulence systems.pCO2represents excesspCO2. (a) Low-turbulence systems (kCO2<1 m d−1). CDOM indirect effect coefficient onfCO2is 0.37, degradation-mediated CDOM indirect effect onfCO2is 0.17.n=102.χ2=5.07,P=0.41, df=5. (b) High-turbulence systems (kCO2>1 m d−1). CDOM indirect effect coefficient onfCO2is 0.39, degradation-mediated CDOM indirect effect onfCO2is 0.30.n=114.χ2=5.45,P=0.24, df=4. Figure 4: The pathways linking CDOM to CO 2 fluxes in high- and low-turbulence systems. Structural equation models linking changes in aquatic CDOM to changes in CO 2 fluxes to the atmosphere for the two subsets of sites separated on the basis of k CO 2 and therefore of average turbulence. Arrows denote directional links between two variables, and the coefficients represent the rate at which a response variable varies as a function of a given change in its predictor, based on centered and standardized data (see Methods). All paths are significant at P <0.001. The dashed arrow denotes a non-significant (NS*) path that was not included in the final model presented here; it is included only for presentation purposes to emphasize the absence of a significant direct link between Pd-DOC and p CO 2 in low-turbulence systems. p CO 2 represents excess p CO 2 . ( a ) Low-turbulence systems ( k CO2 <1 m d −1 ). CDOM indirect effect coefficient on f CO 2 is 0.37, degradation-mediated CDOM indirect effect on f CO 2 is 0.17. n =102. χ 2 =5.07, P =0.41, df=5. ( b ) High-turbulence systems ( k CO2 >1 m d −1 ). CDOM indirect effect coefficient on f CO 2 is 0.39, degradation-mediated CDOM indirect effect on f CO 2 is 0.30. n =114. χ 2 =5.45, P =0.24, df=4. Full size image Collectively, our results highlight the importance of terrestrially derived DOC in fuelling both Bd-DOC and Pd-DOC pools across a wide range of aquatic environments. The variability shown in Fig. 1 suggests that such patterns may have been masked in previous studies conducted at smaller scales or across narrower environmental gradients where autochthonous DOC may have emerged as a more important driver of overall DOC degradability. At the scale of the present study, however, increasing terrestrial influence (as reflected in CDOM) clearly implies higher absolute and relative potentials for DOC to be degraded across lakes, rivers and wetlands. Although those patterns are based on potential degradation rates under standardized conditions, they unambiguously show that both the total amount and the proportion of DOC that can potentially be converted to CO 2 tend to increase with terrestrial influence and, as a corollary, it would be expected that surface water CO 2 concentrations should increase as a function of CDOM. The SEM analyses ( Figs 2 and 4 ) demonstrate that there is a link from CDOM to CO 2 fluxes that is mediated by the degradation of DOC when very large gradients are considered, such that increasing concentrations and subsequent degradation of terrestrial DOC in aquatic ecosystems should indeed result in rising CO 2 emissions. These results, however, do not imply that coloured DOC itself is the only pool being degraded, but rather that systems with high CDOM concentrations are associated with a higher absolute potential for conversion of DOC, both coloured and uncoloured, into CO 2 in surface waters. They do not imply either that DOC degradation is the only factor influencing aquatic CO 2 dynamics in these northern regions. For example, recent inter-regional assessments have highlighted the importance of terrestrial inorganic C inputs in shaping aquatic CO 2 dynamics [6] , [33] , [39] . Similarly, studies that have targeted specific components of the aquatic network, such as low DOC lakes [40] or headwater streams [41] , have also highlighted the importance of soil CO 2 inputs. There is no actual contradiction between these various studies and the results we present here: the direct influence of terrestrial DOC is superimposed onto a background of CO 2 dynamics driven by external inputs of CO 2 . This background is always present but varies both regionally and also locally between different types of aquatic systems [19] , [39] , determined by variations in the relative proportion of DOC versus CO 2 delivered from land to the inland water network. The large heterogeneity that exists among the studied systems was at least partly captured by the SEM analyses performed on subsets of sites sharing comparable patterns in gas exchange coefficient ( Fig. 4 ).When more homogenous sets of systems, in terms of physical structure, were analysed, factors other than DOC degradation emerged as modulating the effect of CDOM on CO 2 concentrations and fluxes. We can only speculate on the causes underlying the differences in pathways linking CDOM to CO 2 in high k CO2 versus low k CO2 systems. It is possible that physical structure integrates other environmental factors that may modulate the impact of CDOM on CO 2 dynamics, such as area and depth [42] , which may in turn be related to residence time, exposure to sunlight or the relative importance of groundwater inputs in regulating CO 2 . Regardless of the actual processes, the different SEM analyses converge to essentially the same conclusion, which remains adequate whether the entire data set or more homogenous subsets of sites are considered. The effect of terrestrially derived DOC on CO 2 evasion is not entirely but significantly driven by DOC processing in continental watersheds. Our results provide a mechanistic underpinning to previous studies that had arrived to similar conclusions concerning the role of DOC but based on regional C mass balances [32] , and also provide a process-based framework underlying the regional relationships that have been observed between DOC concentrations and aquatic CO 2 fluxes [19] , [21] , [22] . We show that DOC degradation strongly mediates this relationship, across rivers ranging from stream order 0 to 6, lakes ranging in size and morphometry from a few hectares to several thousands of square kilometres, and wetlands and ponds that also vary greatly in position and features, within a heterogeneous boreal landscape covering roughly 900,000 km 2 . Our results may not necessarily apply to some specific aquatic components or portions of the landscape but rather provide an integrated perspective of the role of DOC processing in sustaining aquatic CO 2 concentrations and evasion in continental watersheds. The SEM analyses further allow a first-order quantification of the potential effect of shifts in terrestrial DOC concentrations on aquatic f CO 2 . Although the long-term DOC trends are highly variable in time and across landscapes [11] , [12] , [15] , [16] , DOC concentrations have consistently increased across temperate and boreal regions over the past 20 years [7] . More specifically, in our own study area, DOC concentrations have increased between 20 and 50% since 1990 (ref. 43 ), whereas CDOM has increased by up to 155% within the same period in some European landscapes [15] . The coefficients provided by the SEMs ( Fig. 4 ) suggest that for every percent increase in CDOM there should be a 0.17 and 0.30% increase in CO 2 evasion from low and high k CO2 systems, respectively, owing to enhanced DOC processing in those systems. Our results imply that as a consequence, aquatic CO 2 fluxes may have been increasing in northern Québec and elsewhere across northern temperate and boreal landscapes over the past decades, conceivably from 10% to up to 50% where terrestrial DOC concentrations have increased the most. There are, to our knowledge, no long-term data sets on aquatic CO 2 that can be used to test this hypothesis, which we suggest should be incorporated into future long-term research programmes. Our results further suggest that aquatic CO 2 emissions will keep increasing as a direct function of increasing terrestrially derived DOC concentrations in aquatic ecosystems. Considering the major contribution of the aquatic networks in these northern, water-rich landscapes to the global continental aquatic C emissions [1] , [2] , [4] (ca. 1.5 Pg y −1 ), these potential shifts could significantly alter the fine balance that exists between freshwater CO 2 emissions and the estimated continental (2.8 Pg C y −1 ) and oceanic carbon sinks (2.2 Pg C y −1 ) [4] . Although more focused measurements should be undertaken to adequately quantify the magnitude of the enhanced aquatic CO 2 emissions at continental or global scales, the scenario that we propose here undoubtedly involves the mobilization and degradation of terrestrial organic C, which, contrary to historical assumptions, appears to be highly reactive in freshwaters but would otherwise experience much slower degradation in more stable environments such as soil or oceanic refuges [1] , [44] , [45] . The absence of evidence for generalized long-term declines in discharge, and the positive relationships that have been reported between long-term trends in discharge and DOC concentrations in landscapes where browning is happening [11] , [12] , [43] , suggest that greater amounts of DOC are circulating in inland waters today compared with a few decades ago, yet no increase in the export of DOC from continents to the oceans have been observed so far in regions where browning is happening [46] . These observations are consistent with our findings that this additional carbon is readily processed and converted to CO 2 as it enters the aquatic networks, which may further enhance the erosion of the terrestrial C (refs 47 , 48 , 49 ) sink beyond a direct effect of increasing global temperatures. Study area and sampling Over the course of 8 years, we sampled lakes, streams, rivers and wetlands (mostly beaver ponds) located in seven temperate and boreal regions of Québec, eastern Canada (44–53°N, 70–80°W, Supplementary Fig. S5 ). Sites were sampled from late May to early October and a subset of sites was sampled up to three times in a given year. A more detailed description of the regional features can be found in Lapierre and del Giorgio [19] . In short, these regions cover a total area of ~900,000 km 2 and are characterized by a wide range of geography, climate and dominant plant cover: mean annual temperature ranges from 4.9 °C in the Laurentians to −2.0 °C in the Eastmain region, and mean annual precipitations ranges from 695 mm y −1 in the Eastmain to 1,150 mm y −1 in the Eastern Townships regions. Dominant vegetation ranges from deciduous forest in the Eastern Townships and Laurentians regions to mixed deciduous and conifer forest in the Abitibi and Chicoutimi regions; the James Bay, Chibougamau and Eastmain regions are characterized by spruce-moss forest. Topography is generally flat and lakes and rivers are typically shallow and turbid in the low-altitude (typically 200–300 m elevation) Abitibi and James Bay regions, which are located in the Abitibi clay belt. Water discharge was very low in rivers and streams in the latter region, whereas it was the highest in the most elevated and steepest (200–900 m elevation) Laurentians and Chicoutimi regions. Sampling took place from 2003 to 2005 in Eastern Townships, and from 2009 to 2011 in the remaining regions. The Eastern Townships sites were sampled in June, July and August each year, the Eastmain sites were sampled twice from early June to early July 2009, the Laurentians sites were sampled once between mid-June and mid-August 2010, and three sampling campaigns were performed during the ice-free period for the remaining regions in 2010 and 2011. For these latter regions, the first campaign occurred from late May to early June, the second campaign from mid-July to mid-August and the third campaign from late September to early October. A subset of sites were sampled at each campaign and the remaining ones were sampled only once during mid-summer. For this analysis, we have used the indiviudal sampling points, without any averaging. Because of various logistical constraints, not all variables could be measured at every site all the time, which explains the different number of observations presented for the main variables. In addition, DOC photochemical degradability was not measured for the Eastern Townships sites. Water was sampled at 0.5 m from the surface from the deepest measured point of lakes and near the shore of streams, rivers and wetlands. Ambient p CO 2 was measured in situ using an EGM-4 infrared gas analyser (PP-systems, Boston, MA, USA) after equilibration by pumping water through a Liqui-Cel Mini Module (Charlotte, NC, USA) contactor membrane (for lakes) or by headspace equilibrium (rivers, streams and wetlands). Excess p CO 2 was calculated by subtracting ambient atmospheric p CO 2 at the corresponding sites. CO 2 flux, and the associated diffuse gas exchange coefficients for CO 2 ( k CO2 ), were measured for every site on the basis of changes in p CO 2 with time in floating chambers [38] . The chamber was connected in closed loop to an EGM-4 infrared gas analyser (PP-systems), p CO 2 in the chamber was measured every minute for 10 min and accumulation rate was calculated by linear regression. Chemical and optical analyses Coloured dissolved organic matter (CDOM) was determined spectrophotometrically in 0.45-μm filtered natural water samples. We measured absorbance at 440 nm with a ultraviolet–visible Ultrospec 2100 spectrometer (Biochrom, Cambridge, UK) using a 2-cm quartz cuvette and corrected by subtracting nanopure water blanks. The absorption coefficient (a440, in m −1 ) was reported in Naperian units by dividing the optical absorbance at 440 nm by the path length in metres and multiplying by 2.303 (ref. 50 ). Concentrations of DOC from filtered (0.45 μm) water samples were measured in duplicate (taken from a unique vial) on an OI-1010 TIC-TOC Analyzer (OI Analytical, College Station, TX, USA). Total phosphorous ( Supplementary Table S1 ) was analysed spectrophotometrically using the standard molybdenum blue method after persulfate digestion [51] , and Chl a samples ( Supplementary Table S1 ) were analysed spectrophotometrically following filtration on Whatman (Maidstone, UK) GF/F filters and hot ethanol (90%) extraction [52] . Filters were sonicated before extraction. The surface and catchment areas of the lakes we sampled were determined using the ArcView 3.2 and ArcGIS v.9 software applied on the DEM derived from (1:50,000) maps. DOC degradability The DOC degradation data presented here reflect the potential for DOC to be mineralized under standardized conditions, and not to actual degradation rates under ambient conditions. Our approach aimed at removing or minimizing site-specific features such as local temperature and light exposure and thus to ensure that the resulting DOC degradability was comparable across the entire spectrum of sites. Biological degradation experiments were carried out in the dark at a fixed incubation time (14 days) and temperature (20 °C), and the data presented in Fig. 1a thus correspond to the amount of Bd-DOC over a period of 14 days. We filtered 1.5 l of ambient water through 2.7 μm pore-size GF/F filters (Whatman) for biological degradation experiments to preserve most bacteria and avoid re-inoculation [53] . We used the same pool of water for photochemical degradation experiments to minimize the differences in manipulations and thus maximize the comparability of both properties over the large range of samples. Two 500-ml subsamples were used as replicates for biological degradation experiments and dispensed in acid-washed glass bottles (500 ml). Figure 1a presents the average of both replicates. The remainder of the water was used for photochemical degradation experiments, which were carried out in a solar simulator (Qsun XE1-BC, Qlab, FL, USA) under a standard light dose (0.68 W m −2 at 340 nm, spectrum representative of natural sunlight) over a fixed incubation time (24 h) and temperature (24 °C). The data presented in Fig. 1b thus correspond to the amount of photochemically degradable DOC in 1 day at the maximum sustainable light intensity from the solar simulator; considering diel light cycles and the natural light intensity at the studied latitudes, this would roughly correspond to 6 days of natural light exposure in the sampled regions. Irradiated samples were contained in 40 ml glass tubes, and thus the data presented would correspond to loss rates in the first centimetres of the water column. Roughly 80% of the light between 360 and 700 nm passes through the glass, decreasing linearly to reach 10% at 315 nm; no light below 300 nm went through. The measured loss rates are thus conservative compared with what would have been obtained with quartz tubes, but still represent a level of exposure representative of the first centimetres of the water column. Given the very strong light intensity and the small size of the vials, the light dose within the vials was high and the loss rates because of photochemical degradation were high, thus a 24-h period was sufficient to obtain reliable estimates of DOC losses. We assumed that all bacteria were killed by the very high ultraviolet dose. Even if that were not the case, the DOC loss rates owing to photochemical degradation were systematically at least an order of magnitude higher than those measured in the biological degradation experiments (when compared on a per day basis), implying that if bacteria did survive, they could not contribute importantly to the measured loss rates. DOC concentrations were measured within 1 month after incubation. These standardized biological and photochemical degradation rates could potentially be extrapolated to ambient waters by adjusting them for in situ temperature, light exposure and water retention time, among other factors, but this is not the focus of this study. Here we rather concentrate on the comparative analysis of this standardized DOC degradability across sites. Statistical analyses Data were log transformed to attain normality and homoscedasticity. Single regressions were performed using JMP software version 7.0 (SAS Institute, NC, USA). We used major axis (type II) regressions to obtain a representative slope for the regression between two log-transformed variables containing measurement errors in Fig. 1 . We performed SEM to identify the sequences of presumed causal relationships that may exist [37] between CDOM, the amounts of Bd-DOC and Pd-DOC, ambient DOC, excess p CO 2 and f CO 2 , using EQS 6.1 (Multivariate Sofware, CA, USA). This analysis tests the significance of individual paths between variables as well as that of the structure as a whole. Similar to most analyses, a path with P <0.05 is typically considered significant. Regarding the overall model, however, a value of P >0.05 means that the proposed structure effectively captures the variability in the modelled variables and the directional links between them, whereas P <0.05 would imply a significant difference between the observed and the modelled data [37] . The coefficients provided by the SEM for the links between two variables (noted beside the arrows in Figs 2 and 4 ) are conceptually analogous to the slope of the linear regression between those variables, but the computation differs from major axis regressions, thus the coefficients provided by the different types of analyses cannot be directly compared [37] . Furthermore, the log-transformed data have been centred and scaled for the SEM analyses, such that different coefficients within a given structure can be directly compared. A higher coefficient between two variables denotes a stronger link than between two variables linked by a lower coefficient. Further details on the SEM analyses are provided in the Supplementary Note 2 . How to cite this article: Lapierre, J.-F. et al. Increases in terrestrially derived carbon stimulate organic carbon processing and CO 2 emissions in boreal aquatic ecosystems. Nat. Commun. 4:2972 doi: 10.1038/ncomms3972 (2013).